TheOpisthorchis viverrinigenome provides insights into life in the bile duct Opisthorchiasis is a neglected, tropical disease caused by the carcinogenic Asian liver fluke, Opisthorchis viverrini. This hepatobiliary disease is linked to malignant cancer (cholangiocarcinoma, CCA) and affects millions of people in Asia. No vaccine is available, and only one drug (praziquantel) is used against the parasite. Little is known about O. viverrini biology and the diseases that it causes. Here we characterize the draft genome (634.5 Mb) and transcriptomes of O. viverrini, elucidate how this fluke survives in the hostile environment within the bile duct and show that metabolic pathways in the parasite are highly adapted to a lipid-rich diet from bile and/or cholangiocytes. We also provide additional evidence that O. viverrini and other flukes secrete proteins that directly modulate host cell proliferation. Our molecular resources now underpin profound explorations of opisthorchiasis/CCA and the design of new interventions. Parasitic worms (helminths) infect billions of people worldwide and represent a massive socioeconomic burden, similar to diabetes or lung cancer in disability adjusted life years [1] . These worms include roundworms (nematodes) and flatworms (flukes and tapeworms). Foodborne liver flukes (Trematoda: Digenea) cause particularly important, but neglected diseases of humans globally [2] . Opisthorchis viverrini is notable, because it is classified as a group 1 carcinogen by the International Agency for Research on Cancer (IARC) [3] and is a significant risk factor for cholangiocarcinoma (CCA), a deadly cancer of the biliary tree, with a very poor prognosis. Although CCA incidence is low in Western countries, this cancer is prevalent in many parts of South East Asia where O. viverrini is endemic, including northeastern Thailand, Laos and Cambodia, where an age-standardized incidence of up to 96 per 100,000 has been reported [4] . Current estimates indicate that chronic opisthorchiasis affects 10 million people worldwide, and, in Asia, fluke-associated CCA is detected in approximately 2,500 people annually [5] . O. viverrini has a complex life cycle [6] , involving snail and fish intermediate hosts, and piscivorous definitive hosts (including humans, dogs or cats). Humans become infected when they consume raw freshwater fish infected with metacercariae (larval stage), after which the juvenile fluke hatches in the upper small intestine and migrates to the bile ducts, where it develops into a hermaphroditic adult. O. viverrini can live for years in intra- and extra-hepatic bile ducts and the gall bladder. This chronic infection results in cholangitis, fibrosis, cholecystitis, and, in many cases, CCA. Presently, there is no anti- O. viverrini vaccine, and chemotherapy relies on the use of a single drug, praziquantel. However, excessive praziquantel administration can reduce treatment efficacy [7] and induce inflammation of the biliary system [8] . Moreover, even after successful treatment, reinfection with O. viverrini is frequent. Alternative strategies to intervene with O. viverrini infection are thus urgently needed, for instance, by inhibiting pathways in the fluke that are essential for its survival in the bile duct. In this study, we propose that deciphering the O. viverrini genome provides vital insights into the fundamental molecular biology of this parasite, identify essential pathways linked to fluke–host interactions and predict genes that might contribute to CCA tumorigenesis. Knowledge of the O. viverrini genome should also fill critical knowledge gaps in parasite biology, as, to date, most genomic explorations of flukes have focused predominantly on blood flukes (schistosomes) [9] , [10] , [11] , with genome studies of liver flukes still in their infancy [12] , [13] , [14] , [15] . Using Illumina-coupled technology, we generate a high quality draft genome of O. viverrini , and identify key biological and metabolic pathways specific to this parasite that might represent novel targets for intervention. Our de novo assembly should be useful as a reference sequence against which to compare other related metazoan parasites. Genome assembly We produced 79.9 Gb of short-read sequence data, representing ~134-fold genome coverage, from seven genomic DNA libraries constructed from 25 adult O. viverrini specimens. 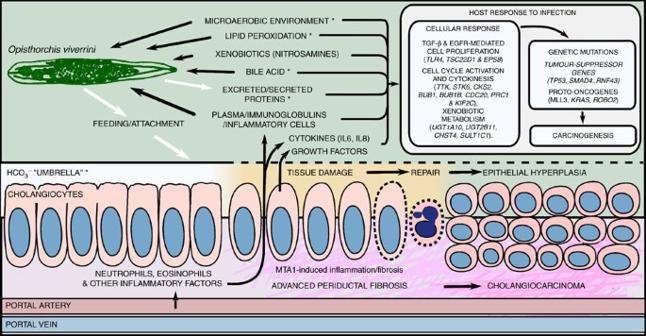Figure 1: Processes proposed to take place during the establishment ofOpisthorchis viverriniin the bile duct and the subsequent pathogenesis of biliary disease and associated cholangiocarcinoma. This proposal integrates salient information from the present study (*) and considers published literature. Metastasis-associated protein 1-mediated fibrosis and transformation of cell cycle progress are linked to: transforming growth factor-beta (TGF-beta) and epidermal growth factor receptor (EGFR)-mediated cell proliferation, associated with an upregulation in Toll-like receptor 4 (TLR4), TGF-beta-stimulated clone 22 homologue (TSC22D1) and EGFR pathway substrate 8 (EPS8); cell cycle activation and cytokinesis associated with an upregulation in dual specificity protein kinase TTK (TTK), serine/threonine kinase 6 (STK6), CDC28 protein kinase regulatory subunit 2 (CKS2), budding uninhibited by benzimidazoles 1 mitotic checkpoint serine/threonine kinase (BUB1 and BUB1B), cell division cycle 20 (CDC20), protein regulator of cytokinesis 1 (PRC1), kinesin family member 2C (KIF2C); and endogenous/exogenous xenobiotic metabolism associated with an upregulation in UDP glucuronosyltransferase 1 family, polypeptide A10 (UGT1A10); UGT 2 family B11 (UGT2B11), carbohydrate sulphotransferase 4 (CHST4) and sulphotransferase family, cytosolic, 1C, member 1 (SULT1C1). Chronic opisthorchiasis is linked to genetic alterations in tumour protein 53 (TP53: 44.4% cases), mothers against decapentaplegic homologue 4 (SMAD4; 16.7%), Kirsten rat sarcoma viral oncogene (KRAS; 16.7%), histone-lysine N-methyltransferase (MLL3; 14.8%), roundabout homologue 2 (ROBO2; 9.3%), guanine nucleotide-binding protein (GNAS; 9.3%) and ring finger protein 43 (RFN43; 9.3%). Library insert sizes ranged from 170 bp to 20 kb ( Supplementary Table 1 ). Based on 17-mer frequency distributions, we consistently found low-sequence heterozygosity within and among short paired-end libraries ( Supplementary Fig. 1 ). 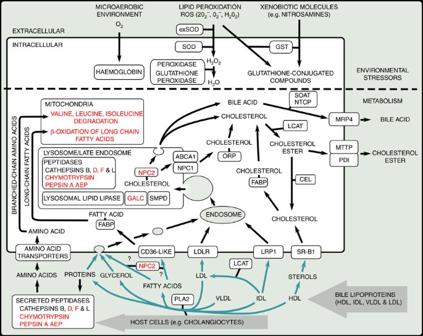Figure 2:Opisthorchis viverrinibiological pathways linked to life in the human bile duct. O. viverrinigenes (boxed) associated with responses to environmental stressors or the processing of abundant nutrients found within the bile duct. Genes unique to opisthorchiids (that is, found inO. viverriniandClonorchis sinensis) or gene families, which have expanded within this group of flukes are shown in red. Pathways required for the degradation and uptake of micelles, including very-low (VLDL), low (LDL), intermediate (IDL) and high density lipoproteins (HDL), are represented by blue arrows. We assembled the genome into scaffolds ( Supplementary Table 2 ), producing a 634.5 Mb draft genome (N50=1,323,951 bp; N90=169,601 bp; longest scaffold: 9,657,388 bp) ( Table 1 ). 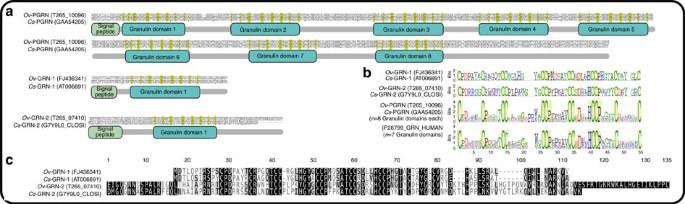Figure 3:Opisthorchis viverriniandClonorchis sinensisproteins with at least one granulin domain. (a) Alignment of the amino acid sequences translated fromO. viverriniandC. sinensisprotein-coding regions of putative progranulin (PGRN) and granulin (GRN-1 and GRN-2) genes, displaying the structural organization of the signal peptide and cysteine-rich granulin domain/s (InterProScan ID: IPR000118). Conserved granulin domain residues are highlighted in yellow. (b) Amino acid logos of conserved granulin domains encoded withinO. viverriniandC. sinensisgranulins (GRN-1 and GRN-2; one granulin domain each), PGRN (eight domains per protein) and human PGRN (seven granulin domains). Logo is coloured on the basis of amino acid chemistry, where amino acid residues are grouped by colour, depending on their chemical characteristics, so that polar residues (G, S, T, Y and C) are green, neutral (Q and N) are purple, basic (K, R and H) are blue, acidic (D and E) are red and hydrophobic (A, V, L, I, P, W, F and M) are black. Residue height denotes the measure of uncertainty for each residue (in bits per symbol). (c) Alignment of the predicted mature opisthorchiid-specific granulin proteins. We detected ~86% of 248 core essential genes, very comparable with ~80–86% for well-assembled trematode genomes ( Supplementary Table 3 ). For O. viverrini , the mean GC content of all genomic scaffolds was 43.7%, similar (44.8%) to the related carcinogenic liver fluke Clonorchis sinensis [13] ( Supplementary Fig. 1 ). A small number of nucleotides ( n =168,414; 0.03%) were subjected to base-calling correction, leading to improved mapping of RNA-seq data ( Supplementary Table 2 ). Table 1 Characteristics of the Opisthorchis viverrini draft genome. Full size table Genome-wide synteny among parasitic flatworms The O. viverrini draft assembly was compared with other fluke genomes to characterize conserved features. First, we compared the O. viverrini genomic scaffolds with those of C. sinensis . Surprisingly, we observed substantial structural variability between these two genomes. Specifically, only 22.0% of O. viverrini scaffolds could be aligned to 25.8% of the C. sinensis scaffolds at the nucleotide level ( Supplementary Table 4 ). We also found limited genomic synteny between O. viverrini and C. sinensis (based on scaffolds of >100 kb). For example, the ten most similar O. viverrini and C. sinensis scaffolds contained 13 syntenic blocks, aligned over 29% and 87% of the C. sinensis and O. viverrini scaffolds, respectively ( Supplementary Table 4 and Supplementary Fig. 2 ). Reciprocally, 63 C. sinensis scaffolds with sequence similarity to a long (~9.7 Mb) O. viverrini genomic scaffold were aligned in 52 syntenic blocks, covering 85% of the O. viverrini scaffold and 48% of the 63 C. sinensis scaffolds. Considerable divergence was also seen when the O. viverrini genome was compared with the blood fluke Schistosoma mansoni . We found that 308 O. viverrini scaffolds with sequence similarity to chromosome 1 of S. mansoni (65,476,681 bp) aligned in 107 syntenic blocks, and covered 35% and 8% of the O. viverrini and S. mansoni scaffolds, respectively ( Supplementary Fig. 2 and Supplementary Table 4 ). Similar divergence was also observed when C. sinensis was compared with S. mansoni ( Supplementary Table 4 ). This lack of synteny likely attributes to differences in karyotype among these flukes. For example, O. viverrini has 2 n =12 chromosomes [16] , whereas C. sinensis has been reported to have 2 n =14 (Russian isolate) [17] or 2 n =58 chromosomes (Korean isolate) [18] ; Schistosoma spp. of humans all have eight chromosomes [19] . These findings indicate that the O. viverrini genome is very divergent from all other fluke genomes published to date [9] , [10] , [11] , [13] . Annotation of noncoding and coding gene regions Our O. viverrini genome provided the basis for the identification and annotation of repetitive and protein-coding elements. Using both similarity-based and de novo prediction methods, we determined that 30.6% of the O. viverrini genome encodes repetitive elements ( Supplementary Data 1 ); this percentage is consistent with C. sinensis (25.6%) [13] , but lower than for Schistosoma spp. (40–47.5%) [9] , [10] , [11] . More than half (61.8%) of the repeats are retrotransposons ( Supplementary Data 1 ), including unclassified, long terminal repeat (LTR) (9.7%), LTR/ Gypsy (8.4%) and LTR/ Pao (0.9%) elements. We also observed a number of long interspersed elements (LINEs), comprising LINE/RTE (23.6%), LINE/CR1 (8.2%) and LINE/ Penelope (5.2%) elements. In total, 16,379 protein-encoding genes ( Table 1 and Supplementary Table 3 ) were predicted from the genome based on transcriptomic evidence from previously published RNA-seq data and sequence similarity to protein-encoding genes of C. sinensis [13] and blood flukes [9] , [10] , [11] . Most genes (14,269; 87.1%) were supported by published RNA-seq data [12] , [15] from both adult and juvenile stages of O. viverrini ( Supplementary Table 1 ), and >99% of de novo -assembled transcripts mapped to the genome. The estimated total number of genes, the proportion of coding regions (3.4%), and the mean total gene length (18,231 bp), intron length (3,531 bp), exon length (254 bp) and mean number of exons per gene (5.8) were similar to those of C. sinensis [13] , but distinct from other flukes ( Supplementary Table 3 ). Both the O. viverrini and C. sinensis genomes exhibit considerable intronic expansions compared with other flukes (mean 2.8–3.5 kb and equating to a 1.2- to 1.5-fold increase in intron length). Noncoding RNA sequence elements were also predicted (806 distinct elements), including tRNAs ( n =189) and conserved microRNAs (178) ( Table 2 ). There was a significant correlation between the frequency of tRNA copies encoded in the genome and amino acid usage in O. viverrini and C. sinensis ( Supplementary Fig. 3 ). The amino acid composition of translated protein-coding domains for these two opisthorchiids was similar to that of fasciolid liver flukes [20] and of tapeworms (cestodes) [21] ( Supplementary Fig. 3 ), suggesting that GC-rich O. viverrini coding domains ( Table 1 and Supplementary Fig. 2 ) encode arginine, alanine, glycine, proline and valine amino acid residues more frequently, and asparagine, isoleucine, serine and tyrosine less frequently than blood flukes ( Supplementary Fig. 3 ). Table 2 Annotation of Opisthorchis viverrini protein-encoding genes and noncoding RNA elements, and their sequence similarity, homology or orthology to predicted protein data sets from other parasitic flatworms that infect humans. Full size table Conserved and O. viverrini -specific pathways The 16,379 O. viverrini protein-coding genes were functionally annotated based on sequence similarity to public sequence, gene ontology (GO) and biological pathway data sets ( Table 2 ). We assigned a subset of the 9,402 genes (57.2%) based on similarity to Kyoto Encyclopedia of Genes and Genomes (KEGG) orthologous gene terms to 184 biological pathways ( Supplementary Data 2 ), and identified O. viverrini genes linked to conserved components of nucleotide, carbohydrate, lipid and amino acid metabolisms, independently confirmed by GO-based analysis ( Supplementary Table 5 ). Cellular processing components, including proteins associated with cell turnover, protein transport and catabolism were also commonly predicted ( Supplementary Table 5 ). We also characterized specific protein classes, including kinases ( n =262), peptidases/proteases (386), glycosyltransferases (84), transcription factors (226), cytoskeletal proteins (212), ion channels (128) and receptors (140), including G protein-coupled receptors (59). Our attention was drawn to peptidases, because many were predicted to be secreted, and might function to degrade extracellular protein complexes and also modulate host immune responses [22] . The O. viverrini peptidases ( n =386) could be divided into five major classes (aspartic, cysteine, metallo-, serine and threonine), with metallo- ( n =168; 43.5%) and serine peptidases ( n =81; 21.0%) predominating ( Supplementary Data 3 ). We also identified multiple copies of secreted aspartic peptidases (for example, cathepsin D; n =27 genes), a large repertoire of cysteine peptidases (cathepsins B, F and L), and a significant expansion of C13-like asparaginyl endopeptidases (AEPs; 94 distinct genes), an observation consistent with transcriptomic data available for this species [12] , [15] . The functional role(s) of AEPs remain unclear, despite a large number of novel members being differentially transcribed between juvenile and adult stages ( Supplementary Data 3 ). These new peptidases might trans-process and activate other peptidases with Asn residues at the point of cleavage between pro- and mature peptidase [23] . Interestingly, members of the large family of O. viverrini cathepsin D peptidases often contain an asparagine at the cleavage site between pro- and mature peptidases. Reflecting their importance in O. viverrini biology, in total, 45 different peptidases are encoded by the top 10% of highly transcribed genes in the juvenile and adult stages inhabiting the biliary tract; these molecules include calpain, a tryptase-like serine peptidase, cathepsin D, F and B, and a C13-like AEP ( Supplementary Data 3 ). We also identified 55 peptidase inhibitors ( Supplementary Data 4 ), of which aspartic (α-2-macroglobulin), serine (α-2-macroglobulin and serpin) and cysteine peptidase inhibitors (cystatins) are enriched in the transcriptome of O. viverrini stages in the biliary tract ( Supplementary Data 4 ). Excretory/secretory (ES) proteins of O. viverrini are likely to be central to fluke–host interactions and contribute to CCA development [24] . We computationally defined an O. viverrini secretome of 437 proteins ( Supplementary Data 5 ); 184 of these molecules (42.1%) shared sequence similarity (BLASTp, E -value ≤10 −5 ) to previously reported ES proteins of O. viverrini and other flukes [24] . Examples of O. viverrini ES proteins include peptidases, heat shock proteins, superoxide dismutase and venom allergen-like proteins ( Supplementary Data 5 ). On a transcription level, ES proteins in the juvenile and adult stages include cysteine peptidases (CatB, AEP), vitelline B, repetin, TP, Niemann-Pick C2 (NPC2) proteins, glutathione-S-transferase (GST), progranulin ( Ov -PGRN) and two opisthorchiid-specific granulins ( Ov -GRN-1 and Ov -GRN-2) ( Supplementary Data 5 ). We then explored similarities in the proteome between O. viverrini and other flukes. Reflecting the genome synteny results ( Supplementary Table 4 ), the 16,379 O. viverrini proteins predicted exhibited the highest degree of sequence similarity (BLASTp, E -value ≤10 −5 ) to those of C. sinensis (13,203; 80.3%), followed by the three human blood flukes ( Schistosoma haematobium, Schistosoma japonicum and S. mansoni ; 9,317–9,377; ~57%) ( Supplementary Fig. 4 ). In total, 8,574 genes were similar among all five fluke species studied; reciprocally, 3,015 genes (18.3%) were unique to O. viverrini relative to the other four flukes. Considering significant differences in global, pairwise sequence similarity among key flukes and tapeworms ( Supplementary Fig. 5 ), OrthoMCL was used to further cluster proteins; 5,160 conserved orthologs were shared among all eight flatworm species ( Supplementary Fig. 4 ). Using the OrthoMCL clusters, we also identified orthologous groups in the opisthorchiids O. viverrini and C. sinensis ( n =2,037) that have diverged with respect to blood flukes and tapeworms; 1,941 of these genes represented single-copy, one-to-one orthologues ( Table 2 and Supplementary Table 6 ), and included proteins linked to differences in developmental body plan and in nutritional sources used by different parasitic flatworms. Conspicuous were O. viverrini proteins involved in cytoskeletal microtubule-mediated organelle transport and centrosome assembly (dyneins and kinesins); transcription repressors (Krüppel-associated box domain-containing zinc finger proteins) and enhancers (GATA-binding proteins and SOX 1/2/3/14/21) regulating sex determination and other gene regulatory networks involved in developmental progression [25] ; and ubiquitin-protein ligases binding to specific protein substrates, catalysing the transfer of ubiquitin and signalling protein degradation or other protein–protein interactions [26] . Metabolic enzyme families have also evolved in opisthorchiid flukes, including peptidases that likely function in feeding (such as cathepsin D and pepsin A) and cell movement (leishmanolysin-like peptidases), and glycosyltransferases that participate in the glycosylation of secretory proteins (glycoprotein-N-acetylgalactosamine 3-beta-galactosyltransferases and alpha-1,6-mannosyl-glycoprotein 6-beta-N-acetylglucosaminyltransferases) and glycosphingolipid biosynthesis (N-acetyllactosaminide beta-1,6-N-acetylglucosaminyl-transferase; Supplementary Table 7 ). Among all opisthorchiid orthologous protein groups, 212 were predicted as ES proteins, including 143 proteins predicted for O. viverrini specifically ( Supplementary Data 5 ). Among them are granulins, which are implicated in carcinogenesis in humans [27] , and other proteins inferred to be involved in parasite–host interactions, including venom allergen-like (VAL) proteins [22] and cathepsin L [28] ( Supplementary Data 5 ). Further study of these orthologous groups should reveal adaptations of opisthorchiids to their unique environment in their intermediate (snail) and definitive (human) hosts. Evolutionary adaptations to life in the biliary system We sought to relate features of the O. viverrini genome to its unique biology. We focused specifically on the migration of the fluke to and survival in the bile duct, and the absorption, binding and conversion of nutrients within the biliary system ( Fig. 1 ). Figure 1: Processes proposed to take place during the establishment of Opisthorchis viverrini in the bile duct and the subsequent pathogenesis of biliary disease and associated cholangiocarcinoma. This proposal integrates salient information from the present study (*) and considers published literature. Metastasis-associated protein 1-mediated fibrosis and transformation of cell cycle progress are linked to: transforming growth factor-beta (TGF-beta) and epidermal growth factor receptor (EGFR)-mediated cell proliferation, associated with an upregulation in Toll-like receptor 4 (TLR4), TGF-beta-stimulated clone 22 homologue (TSC22D1) and EGFR pathway substrate 8 (EPS8); cell cycle activation and cytokinesis associated with an upregulation in dual specificity protein kinase TTK (TTK), serine/threonine kinase 6 (STK6), CDC28 protein kinase regulatory subunit 2 (CKS2), budding uninhibited by benzimidazoles 1 mitotic checkpoint serine/threonine kinase (BUB1 and BUB1B), cell division cycle 20 (CDC20), protein regulator of cytokinesis 1 (PRC1), kinesin family member 2C (KIF2C); and endogenous/exogenous xenobiotic metabolism associated with an upregulation in UDP glucuronosyltransferase 1 family, polypeptide A10 (UGT1A10); UGT 2 family B11 (UGT2B11), carbohydrate sulphotransferase 4 (CHST4) and sulphotransferase family, cytosolic, 1C, member 1 (SULT1C1). Chronic opisthorchiasis is linked to genetic alterations in tumour protein 53 (TP53: 44.4% cases), mothers against decapentaplegic homologue 4 (SMAD4; 16.7%), Kirsten rat sarcoma viral oncogene (KRAS; 16.7%), histone-lysine N-methyltransferase (MLL3; 14.8%), roundabout homologue 2 (ROBO2; 9.3%), guanine nucleotide-binding protein (GNAS; 9.3%) and ring finger protein 43 (RFN43; 9.3%). Full size image O. viverrini migration to and establishment in the bile duct. When ingested by the human host, metacercariae of O. viverrini pass through the alimentary tract, where they excyst, migrate to the sphincter of Oddi and then establish within the biliary tract [29] . Some peptidases, including aspartic and cysteine peptidases, likely have a key role in initiating excystment ( Supplementary Data 3 ) and are highly transcribed in opisthorchiid metacercariae [14] . The large number of GPCRs and ion channels present in O. viverrini ( Supplementary Data 2 and Supplementary Table 8 ) could enable chemotaxis-mediated migration to the biliary duct, including the rhodopsin biogenic amine receptors and ion channels, which are conserved in opisthorchiids, but divergent from homologues in other parasitic flukes that live outside the biliary system (see Supplementary Table 7 ). Survival in an inhospitable environment. Oxygen levels in the human bile duct can vary considerably and are often low, particularly in patients with cholecystitis [30] . Therefore, fluke haemoglobin, with its exceptionally high oxygen affinity [31] , is linked to high transcription in O. viverrini within the bile duct ( Fig. 2 and Supplementary Data 6 ). Like other flukes [32] , O. viverrini is a facultative anaerobe, within the bile duct, transcribing genes associated with anaerobic (including phosphoenolpyruvate carboxykinase) and aerobic (such as pyruvate kinase) glycolysis ( Supplementary Data 6 ) [33] . Figure 2: Opisthorchis viverrini biological pathways linked to life in the human bile duct. O. viverrini genes (boxed) associated with responses to environmental stressors or the processing of abundant nutrients found within the bile duct. Genes unique to opisthorchiids (that is, found in O. viverrini and Clonorchis sinensis ) or gene families, which have expanded within this group of flukes are shown in red. Pathways required for the degradation and uptake of micelles, including very-low (VLDL), low (LDL), intermediate (IDL) and high density lipoproteins (HDL), are represented by blue arrows. Full size image Bile induces cellular stress through the generation of free oxygen radicals via lipid peroxidation [34] , and biliary duct cells are frequently exposed to liver-derived endogenous and exogenous toxins, carcinogens, drugs and their metabolites (xenobiotics) [35] ( Fig. 2 ). Within the bile duct, O. viverrini protects its cells through a repertoire of antioxidants ( Supplementary Data 6 ), reflected in highly transcribed intra- and extra-cellular SODs, which can convert free radicals to hydrogen peroxide, glutathione-S-tranferases, which protect the parasite by reducing lipid hydroperoxides [36] , and detoxifying xenobiotic substrates via glutathione conjugation [35] . Indeed, secretory GSTs are expressed in opisthorchiids in response to human bile [37] . Like other flukes [38] , O. viverrini lacks catalases, and relies on peroxiredoxin- and glutathione-like peroxidases to convert hydrogen peroxide to water, reflected in a high transcription of these genes in this parasite within the bile duct ( Supplementary Data 6 ). Evading the host immune system. Evasion of the host immune response is of paramount importance, particularly if inflammation ensues from cellular damage caused by fluke feeding and/or attachment. The present data indicate that ES proteins modulate the host immune response. For instance, genes encoding secreted O. viverrini helminth defence proteins (for example, T265_13308) are highly transcribed in bile duct stages ( Supplementary Data 6 ). In other flukes, these proteins are proposed to mimic the mammalian host defence peptide (called cathilicidin) and subvert a Th1 response by preventing the interaction of LPS with the Toll-like receptor 4 complex on macrophages [39] . In addition, cathepsin F peptidases of O. viverrini likely degrade immunoglobulins, including the key, secretory immunoglobulin A [40] . Homologous proteins in O. viverrini might have similar immuno-modulatory functions and warrant detailed experimental study. Food and energy sources. The newly excysted juvenile stage of O. viverrini relies initially on energy stored within glycogen granules and lipid droplets in the excretory bladder of the worm [41] . However, once in the bile duct, these energy reserves rapidly deplete, and the developing fluke must acquire food and energy resources essential for growth, development and reproduction. Soaked in bile, O. viverrini can use large amounts of lipoprotein metabolites. Specifically, bile is rich in micelles, high, intermediate, low and very-low density lipoproteins, which are composed of varying proportions of triglycerides, phospholipids, cholesterol and amphipathic proteins [42] . Bile is also rich in branched-chain amino acids [43] and long-chain saturated palmitic acid (C16:0) as well as unsaturated linoelaidic (C18:2) and arachidonic (C20:4) fatty acids [44] . In contrast, although O. viverrini uses glycolysis for energy production, bile is usually depleted of glucose [45] ; thus, this fluke has evolved several adaptations to a life in bile ( Fig. 2 ). Both juvenile and adult stages established in the bile duct transcribe genes encoding enzymes and accessory proteins directly involved in processing bile constituents, including the degradation of free lipids (via mitochondrial fatty acid beta-oxidation) and proteins (via branched-chain amino acid metabolism; Supplementary Fig. 6 ). Notably, these genes are also present in C. sinensis , but are absent from blood flukes and tapeworms, reflecting the lipoprotein-rich environment within the bile duct ( Supplementary Fig. 6 and Supplementary Data 6 ). Interestingly, we identified phospholipases, including an orthologue of C. sinensis secreted phospholipase A2 (PLA2) [46] . These lipases can initiate the degradation of stable micelles and possibly also host cell membranes [47] , to enhance carbohydrate, lipid and protein availability to the fluke. In addition, O. viverrini produces a vast array of enzymes and accessory proteins needed to further degrade micelles ( Fig. 2 ). Examples include cysteine (cathepsins F and B and AEPs), serine (chymotrypsin-like) and aspartic (pepsin-like and cathepsin D) ES peptidases, which are transcribed in these developmental stages (see Supplementary Data 6 ). Collectively, these peptidases offer broad substrate specificity, and might degrade other lipoprotein complexes and proteins. Once degraded, the transfer of free, bile-derived amino acids into tissues and cells of O. viverrini is likely to occur via amino acid transporters ( Fig. 2 and Supplementary Data 6 ), which are then processed for energy production via acetyl CoA ( Fig. 2 ). O. viverrini is unable to synthesize cholesterol de novo. As an alternative, O. viverrini has evolved key molecular pathways to acquire, transport and process cholesterol from the external lipid-rich environment within the bile duct ( Fig. 2 ). This fluke transcribes a homologue of the scavenger-like receptor (SR-B1), which transports cholesterol from HDLs across plasma membranes [48] . It also uses proteins homologous to the LDL receptor (LDLR), LDLR-related protein 1 receptor (LRP1) and CD36-like receptors to facilitate LDL, IDL and fatty acid uptake, respectively ( Supplementary Data 6 ). Within the late endosome and lysosomal compartments, cholesterol esters are hydrolysed to free cholesterol via an acid lipase ( Fig. 2 and Supplementary Data 6 ). To avoid an accumulation in lysosomes in the fluke, cholesterol might be bound to one NPC2-like protein and transported into the cytosol via the Niemann-Pick C1 and adenosine triphosphate-binding cassette transporter 1 complex [49] . Here, once bound to oxysterol-binding protein-related proteins, cholesterol can be transferred to the cytosol, where it is converted to a cholesterol ester by lecithin:cholesterol acyltransferase for subsequent elimination from O. viverrini cells via an MTTP/PDI-like complex. O. viverrini also transcribes genes associated with the molecular transfer of endocytosed bile acids. For instance, bile acids might be transported, via sodium-dependent organic anion transporters (NTCP and SOAT), out of cells using a homologue of multidrug resistance protein MRP4, a signal peptide domain-binding cassette superfamily member which, in humans, mediates an adenosine triphosphate-dependent unidirectional efflux of organic anions from hepatocytes [50] . Strikingly, we also identified a massively expanded family of 25 lipid-binding proteins in O. viverrini and C. sinensis ( Supplementary Fig. 7 and Supplementary Data 6 ); these proteins contain a conserved MD-2-related lipid-binding domain and are homologous to the human NPC2 protein [51] , which operates to facilitate intracellular and extracellular sterol transport [51] . Remarkably, other eukaryotes studied to date appear to have only one copy of this NPC2-like protein [51] . Of the 25 O. viverrini NPC2-like proteins, 15 were transcribed in developmental stages within the bile duct ( Supplementary Fig. 7 and Supplementary Data 6 ). The expansion of this family reflects the importance of the binding and transportation of sterols and/or lipids, including the intracellular transportation of cholesterol in O. viverrini ( Fig. 2 ). Interestingly, in addition to the adaptation of O. viverrini to a lipid-rich diet, our findings ( Fig. 2 and Supplementary Data 6 ) also support the hypothesis that this fluke can digest cholangiocytes. Specifically, O. viverrini juveniles and adults transcribe genes of an opisthorchiid-specific galactosylceramidase/galactocerebrosidase and sphingomyelin phosphodiesterases ( Fig. 2 and Supplementary Data 6 ). In the lysosome, these enzymes are essential for catabolising sphingomyelin, a highly enriched constituent of cholangiocytes [52] . In conclusion, O. viverrini transcribes genes encoding an extensive repertoire of enzymes and receptors required for the absorption, binding and/or conversion of nutrients originating almost exclusively from the bile and biliary epithelium. Such adaptations likely permit O. viverrini to effectively use the salient constituents of bile and biliary epithelium to survive under extremely harsh physiological conditions within the biliary tract. Role of O. viverrini in CCA development Chronic O. viverrini infection is a major risk factor for CCA [8] . Exome sequencing of CCAs from patients with known O. viverrini infection suggests a multifactorial aetiology [53] , with genetic alterations in tumour suppressor genes as well as proto-oncogenes ( Fig. 1 ). In Thailand, factors contributing to an accumulation of genomic and epigenomic alterations in cholangiocytes include: (i) exogenous carcinogens, such a nitrosamines, known to be present in diets rich in fermented fish (‘pla-ra’) and pork [54] ; (ii) fibrosis linked to a metastasis-associated protein 1 and an interleukin-6 (IL-6)-regulated chronic inflammatory response to infection [55] , [56] ; (iii) cell damage or cell death linked to O. viverrini feeding and/or attachment [8] ; and (iv) transforming growth factor-beta (TGF-beta) and/or epidermal growth factor (EGF)-mediated cell proliferation associated with an extensive repertoire of ES molecules from O. viverrini [57] . Various mechanisms have been proposed to explain how O. viverrini infection contributes to CCA. For example, host inflammation caused by cell damage or cell death, linked to parasite feeding and/or attachment, likely contributes to tumorigenesis ( Fig. 1 ). The biliary epithelium protects underlying cells, including hepatocytes, from the detergent effect of bile acids and from a loss of lipids by maintaining high concentrations of cholesterol and sphingomyelin in the luminal (apical) membrane of cholangiocytes [52] . A protective umbrella of bicarbonate (HCO 3 − ) from these cells provides additional protection from deprotonated bile acids [58] . Damage to this interface can lead to chronic exposure of cholangiocytes to conjugated bile acids that can induce the expression of inflammatory mediators (that is, IL-6 and IL-8), leading to increased oxidative stress and DNA damage, and subsequent fibrosis and tumorigenesis [59] . Micelle degradation by O. viverrini might also accelerate the release of bile acids, which would exacerbate these pathogenic effects. In addition, recent evidence suggests that O. viverrini secretes proteins that directly modulate host cell proliferation. These include a secreted, mitogenic, granulin-like growth factor ( Ov -GRN-1), which is highly transcribed in both juveniles and adults of O. viverrini ( Supplementary Data 6 ). Motivated by this finding, we explored the O. viverrini genome for other potential stimulatory molecules. We identified O. viverrini progranulin ( Ov -PRGN) ( Supplementary Fig. 6 ), required for endogenous regulation of cell growth, development and maintenance [60] . Interestingly, we also identified a novel single-domain, ES granulin ( Ov -GRN-2), which is transcribed in both juvenile and adult stages ( Fig. 3 and Supplementary Data 6 ); PGRN and Ov -GRN-1 and -2 orthologues were also identified in C. sinensis . Comparative sequence analyses of opisthorchiid pro-granulins and granulins identified a conserved granulin domain, CX 6 CX 6 CCX 4–5 GX 3–5 CCPX 5 CCXDX 2 HCCPX 4 CX 5–6 C, predicted to form a stack of four beta hairpins [61] . Overall, Ov -GRN-1 and Ov -GRN-2 share most sequence homology to the granulin domains of Ov -PRGN and its human ortholog ( Fig. 3 ). Although the function of Ov -GRN-2 remains to be determined, differences in the amino acid sequence in the N- and C-termini indicate variation in granulin receptor-binding specificity [60] . Given the known agonistic and antagonistic regulations of cell growth by human granulins [60] , future studies should explore the mitogenic potential of Ov -GRN-2 vis-à-vis Ov -GRN-1. In this context, consideration should also be given to the oncogenic potential of the large family of secreted cathepsin D peptidases ( Supplementary Data 6 ), which can also function as mitogens. In humans, cathepsin D is known to act as a growth factor for several cancers via the proteolytic degradation of growth regulators, growth factor receptors and extracellular matrix components [62] . Figure 3: Opisthorchis viverrini and Clonorchis sinensis proteins with at least one granulin domain. ( a ) Alignment of the amino acid sequences translated from O. viverrini and C. sinensis protein-coding regions of putative progranulin (PGRN) and granulin (GRN-1 and GRN-2) genes, displaying the structural organization of the signal peptide and cysteine-rich granulin domain/s (InterProScan ID: IPR000118). Conserved granulin domain residues are highlighted in yellow. ( b ) Amino acid logos of conserved granulin domains encoded within O. viverrini and C. sinensis granulins (GRN-1 and GRN-2; one granulin domain each), PGRN (eight domains per protein) and human PGRN (seven granulin domains). Logo is coloured on the basis of amino acid chemistry, where amino acid residues are grouped by colour, depending on their chemical characteristics, so that polar residues (G, S, T, Y and C) are green, neutral (Q and N) are purple, basic (K, R and H) are blue, acidic (D and E) are red and hydrophobic (A, V, L, I, P, W, F and M) are black. Residue height denotes the measure of uncertainty for each residue (in bits per symbol). ( c ) Alignment of the predicted mature opisthorchiid-specific granulin proteins. Full size image Chronic opisthorchiasis of humans is associated with extensive damage to the hepatobiliary system, which predisposes to CCA [8] . The cause of this cancer is multifactorial, but clearly linked to O. viverrini in the biliary tract, particularly its attachment, metabolites produced and ES molecules. In geographical regions in which O. viverrini is highly endemic, the age-standardised incidence of CCA in humans can be up to 37-fold greater than that in non-endemic areas [63] . Because there is no effective drug against CCA, and because the culture of eating raw fish is entrenched in areas endemic for opisthorchiasis [54] , intervention relies solely on treatment with the drug praziquantel. Given the potential for drug resistance to develop, there is a major need to find alternative methods of treatment and control, built on a profound understanding of the biology of the parasite and the interplay between the parasite and its hosts at the molecular and biochemical levels. The present study provides the first global insight into the biology of O. viverrini during its establishment in and its adaptation to a life in an inhospitable environment within the bile duct. The molecular findings provide exciting prospects to elucidate the pathogenesis of the opisthorchiasis/CCA complex, and to gain unique insights into why O. viverrini is so pervasive in its human host. Improved understanding of the unique biochemical pathways in O. viverrini linked to its evolutionary adaptation to a bile-rich environment should facilitate the identification of useful intervention targets against the parasite, assisted also by comparative genomic/transcriptomic analyses to identify essential genes and gene products. Essentiality can now be validated using tools such as RNA interference [64] and/or CRISPR RNA-guided Cas9 nuclease-based genome editing [65] . The genomic and transcriptomic resources for O. viverrini should also facilitate urgently needed proteomic, glycomic, lipidomic and metabolic explorations of this and related flukes. From a broader perspective, the O. viverrini genome should underpin detailed investigations of the population genetics and molecular epidemiology of this parasite, and support comparative explorations of related, neglected tropical diseases [1] . The revolution in omics and advanced informatics technologies, combined with the availability of an increasing number of annotated helminth genomes, provides an impetus for rapid progress in fundamental and applied research of neglected tropical diseases, affecting hundreds of millions of people in impoverished regions of the world, in the spirit of the 2012 London Declaration [66] . Production and procurement of parasite material Metacercariae of O. viverrini were isolated from naturally infected fish (including Puntius altis, Prochilodus brevis and Hampala dispar ; Cyprinidae) from a highly endemic region (Ban Pai) in Khon Kaen province, Thailand, using an established method [67] . Helminth-free Syrian golden hamsters ( Mesocricetus auratus ; family Cricetidae) were each infected by gastric gavage with 50 metacercariae [67] . This experiment was approved by the Khon Kaen University animal ethics committee. After 8 weeks, hamsters were euthanized with ether, and the adult worms expressed from the livers (bile ducts), incubated in vitro [12] to allow the worms to regurgitate contents from the alimentary tract, and then washed extensively in physiological saline, snap-frozen in liquid nitrogen and stored at −80 °C until use. Genome sequencing and data processing High molecular weight genomic DNA (>15 kb; ~9.6 μg) was isolated from 25 adult O. viverrini . The amount of DNA was determined using a Qubit fluorometer dsDNA HS Kit (Invitrogen), and DNA integrity verified by agarose gel electrophoresis. Subsequently, short-insert (170, 500 and 800 bp) and mate-paired (2, 5, 10 and 20 kb) genomic DNA libraries were constructed, and paired-end sequenced conducted using TruSeq sequencing chemistry utilizing the HiSeq2000 sequencing platform (Illumina). Whole-genome amplification, using the REPLI-g Midi Kit (Qiagen), was used to produce adequate amounts (>20 μg) of genomic DNA for the construction of all three mate-paired libraries. The sequence reads produced from each library were verified, and low quality sequences, base-calling duplicates and adaptors removed. Sequences from short-insert libraries were error-corrected after establishing a k -mer (=17) frequency distribution [68] . Briefly, sequences were removed if >10% bases were ambiguous (represented by the letter N) or multiple adenosine monophosphates (poly-A), and all remaining reads were filtered based on Phred quality. For sequence data derived from small-insert libraries (that is, 170, 500 and 800 bp), individual reads were removed if >65% of their bases had a Phred quality of <8. For sequence data derived from large-insert libraries (2, 5, 10 and 20 kb), individual reads were removed if >80% of their bases were of this quality. Before assembly, the level of heterozygosity within the population of adult worms of O. viverrini used for sequencing was estimated by establishing the frequency of occurrence of each 17 bp k -mer [68] within the sequence data representing all small-insert libraries. Genome assembly Paired-end sequence data produced from the genomic DNA libraries were assembled in two stages. Initially, using SOAPdenovo ( http://soap.genomics.org.cn/soapdenovo.html ), contigs were assembled from sequence reads from all short-insert libraries, employing a k -mer value of 35; then, contigs were scaffolded using all paired-end reads (produced from short-insert and 2 to 10 kb mate-paired libraries), with ≥3 read pairs being required to form a connection. Assembled sequences were then re-scaffolded and gaps closed using 20 kb mate-paired libraries and additional genomic DNA sequence data (200 and 5,500 bp insert-size libraries) generated from an isoline of F2 O. viverrini progeny (200 flukes) maintained at Khon Kaen University, Thailand, employing the programs Opera ( http://sourceforge.net/projects/operasf/ ) and GapCloser ( http://soap.genomics.org.cn/soapdenovo.html ). Genomic regions containing insertion/deletion and assembly errors were corrected using the program PAGIT iCORN ( http://www.sanger.ac.uk/resources/software/pagit/ ) employing reads from the 800 bp genomic DNA library. The quality of the genomic assembly was assessed by establishing the frequency of nucleotide mismatches between published RNA sequence data and genome scaffolds before and after iCORN correction. Single-end Illumina RNA-seq data from juvenile (2 weeks old) and adult (8 weeks old) O. viverrini [15] were mapped to the genomic scaffolds using TopHat ( http://tophat.cbcb.umd.edu/ ) employing default settings, and reads that mapped to individual scaffolds were collated using SAMtools ( http://samtools.sourceforge.net/ ). For Roche 454 RNA sequence data from adult (8-week-old) O. viverrini [12] , reads that mapped to genomic scaffolds using BLAT ( http://genome.ucsc.edu ) were retained if they aligned perfectly over 200 bases or more. The completeness of the final draft genome assembly and the presence and redundancy of conserved eukaryotic genes in the final scaffolds were assessed using the program CEGMA ( http://korflab.ucdavis.edu/datasets/cegma/ ). In addition, the quality of the assembly and nucleotide accuracy were assessed by aligning all filtered reads to the scaffolds using Burrows–Wheeler Aligner ( http://bio-bwa.sourceforge.net/ ); sequencing depth was estimated by mapping reads to individual scaffolds, and GC content assessed based on a frequency distribution of these data. The GC content of the genomic scaffolds was estimated using a customized Perl script, employing 1 kb nonoverlapping sliding windows. All sequence data can be downloaded from http://bioinfosecond.vet.unimelb.edu.au/Opisthorchis_viverrini/Opisthorchis_viverrini_data.html and National Center for Biotechnology Information (NCBI; BioProject: PRJNA222628). Genome-wide synteny The genome of O. viverrini was compared, in a pairwise manner, with the published draft genomes of C. sinensis (from China) [13] and/or S. mansoni (Puerto Rican strain) [11] . Genomic scaffolds were aligned using the nucmer (nucleotide similarity) or promer (amino acid similarity) tools within the program MUMmer ( http://mummer.sourceforge.net/ ) to assess genome-wide similarities. Subsequently, synteny was explored among three sets of sequence data: (a) O. viverrini and C. sinensis scaffolds (>1,000 bases) that aligned, at the amino acid level, with S. mansoni chromosome 1 (65,476,681 bases); (b) C. sinensis scaffolds that aligned, at the amino acid level, with the largest O. viverrini scaffold (scaffold 1; 9,657,388 bases); and (c) the 10 most similar C. sinensis and O. viverrini scaffolds, based on nucleotide sequence alignment. Conserved syntenic blocks within scaffolds were identified and displayed using the program SyMap ( http://www.agcol.arizona.edu/software/symap/ ). Identification and annotation of repeat and noncoding elements The frequency of interspersed repeat sequence elements within the O. viverrini genome was assessed. Repetitive elements were predicted ab initio using the programs RepeatModeler (v.1.0.4; http://www.repeatmasker.org/RepeatModeler.html ), PILER ( http://drive5.com/piler/ ) and LTR_FINDER ( http://tlife.fudan.edu.cn/ltr_finder/ ). All of these elements were merged into a non-redundant, ‘consensus repeat database’ for O. viverrini . In the genome, simple repeats, satellites and low complexity repeats as well as consensus repeat sequences and those similar in sequence to those in the Repbase library (release 17.02; http://www.girinst.org/server/RepBase/ ) were annotated using RepeatMasker ( http://www.repeatmasker.org/ ). Transfer RNA (tRNA) genes in the O. viverrini genomic scaffolds were predicted using the program tRNA-scan-SE ( http://lowelab.ucsc.edu/tRNAscan-SE/ ) employing default parameters and selecting tRNA-like elements with a predicted covariance model score of >50 (ref. 69 ). Conserved microRNAs and small noncoding nRNAs were predicted using the program INFERNAL (v.1.1rc2; http://infernal.janelia.org/ ) against the Rfam database (release 11.0; http://rfam.sanger.ac.uk/ ). Identification and annotation of protein-encoding genes The protein-encoding gene set of O. viverrini was inferred using de novo -, similarity- and evidence-based approaches. First, assembled juvenile (2-week-old) and adult (8-week-old) transcriptomic sequence data [12] , [15] were examined for predicted full-length ORFs (with predicted start and stop codons) using customized python scripts. These ORFs were then used to train the de novo gene prediction programs SNAP ( http://korflab.ucdavis.edu/software.html ) and AUGUSTUS ( http://augustus.gobics.de/ ). In addition, all raw reads representing the combined O. viverrini transcriptome were used to explore transcript diversity and exon–intron boundaries using the programs TopHat and Cufflinks ( http://cufflinks.cbcb.umd.edu/ ). A consensus gene set for O. viverrini was predicted using the program MAKER2 ( http://www.yandell-lab.org/software/maker.html ), employing evidence of gene-like elements derived from full-length ORFs predicted from the assembled transcriptomic sequence data [12] , [15] , de novo gene predictions using SNAP ( http://korflab.ucdavis.edu/software.html ) and AUGUSTUS ( http://augustus.gobics.de/ ), and utilizing conceptually translated proteins inferred from gene sets for the flukes C. sinensis [13] , S. haematobium [9] , S. japonicum [10] and S. mansoni [11] . Genes inferred to encode peptides of ≥30 amino acids in length were preserved. The gene set was filtered to remove sequences that shared similarity to transposable elements (see Section Identification and annotation of repeat and noncoding elements in the genome). In addition, any genes with identity at the nucleotide (E-value≤10 −5 ) and inferred protein (E-value ≤10 −50 ) levels to those of known microbial organisms were excluded. Finally, the non-redundant gene set of O. viverrini was shown not to contain any Syrian golden hamster (host) DNA by performing a nucleotide sequence search against the genome of the Chinese hamster ( Cricetulus griseus ; family Cricetidae), for which extensive data exist ( http://www.ncbi.nlm.nih.gov/nuccore/?term=txid10029 ). To assess the quality and accuracy of the final gene set predicted, the length distribution of all genes and coding sequences (CDS), the GC content of CDS, exon and introns, and the distribution of exon numbers for individual genes were established, and then compared with values calculated for the published gene sets of C. sinensis , S. mansoni , S. japonicum and S. haematobium [9] , [10] , [11] , [13] . The GC content of the CDS was estimated using 100 bp nonoverlapping sliding window analysis. To infer gene transcription levels, single-end Illumina RNA-seq data from juvenile (2 weeks old) and adult (8 weeks old) O. viverrini [15] were mapped to CDS using the Burrows–Wheeler Aligner ( http://bio-bwa.sourceforge.net/ ) employing default settings and collated using SAMtools ( http://samtools.sourceforge.net/ ). ; the numbers of mapped reads were normalized for length (that is, reads per kilobase per million reads) [70] . For individual genes, a relative measure of transcription was inferred by ranking reads per kilobase per million reads values (highest to lowest): the top 25% of genes were defined as having high transcription, 26–75% as medium and 75–100% as low. Functional annotation of all predicted protein sequences First, following the prediction of the protein-encoding gene set for O. viverrini, each inferred amino acid sequence was assessed for conserved protein domains using the program InterProScan ( http://www.ebi.ac.uk/Tools/pfa/iprscan/ ) employing default settings. Based on their sequence similarity to conserved domains and protein families, proteins inferred for O. viverrini were classified individually according to GO categories and assigned parental (that is, level 2) terms ( http://www.geneontology.org/ ). Second, amino acid sequences were subjected to BLASTp ( E -value ≤10 −5 ) against the following protein databases for C. sinensis [13] , S. haematobium [9] , S. japonicum [10] and S. mansoni [11] ; Swiss-Prot and TrEMBL within UniProtKB ( http://www.uniprot.org/ ); G protein-coupled receptors (GPCRs) and Kinase SARfari ( https://www.ebi.ac.uk/chembl/sarfari/gpcrsarfari and https://www.ebi.ac.uk/chembl/sarfari/kinasesarfari ); KEGG ( http://www.genome.jp/kegg/ ); NCBI non-redundant protein database ( http://www.ncbi.nlm.nih.gov/ ); transporter classification database ( http://www.tcdb.org/ ). Finally, the BLASTp results were used to infer key protein groups, including peptidases, kinases, phosphatases, GTPases, GPCRs, channel and transporter proteins, and transcription factors. Each protein-encoding gene was assigned to a KEGG orthologous gene group using KOBAS ( http://kobas.cbi.pku.edu.cn/home.do ). Individual genes linked to a KEGG orthologous gene term were assigned to known protein families and biological pathways using the KEGG BRITE and KEGG PATHWAY hierarchies using custom scripts. Putative signal peptide and transmembrane domains were predicted using the program Phobius ( http://phobius.sbc.su.se/ ). Classical ES proteins were inferred based on the presence of signal peptide domains and the absence of transmembrane domains. The cellular location of each putative O. viverrini ES protein was then predicted using MultiLoc2 ( http://abi.inf.uni-tuebingen.de/Services/MultiLoc2 ). The final set of ES proteins included only molecules predicted to be transported to the extracellular environment or that shared sequence similarity to proteins within a curated database of validated ES proteins representing O. viverrini or other flukes [9] . In the final annotation, proteins inferred from genes were classified based on their similarity (BLASTp, E -value ≤10 −5 ) to sequences in (a) a curated ES protein database [9] , (b) the KEGG database, (c) Swiss-Prot database and (d) a recognized, conserved protein domain based on InterProScan analysis. Any inferred proteins without a match ( E -value ≤10 −5 ) in at least one of these databases were designated hypothetical proteins. The final protein-encoding gene set for O. viverrini is available for download via the NCBI Bioproject PRJNA222628 or via http://bioinfosecond.vet.unimelb.edu.au/Opisthorchis_viverrini/Opisthorchis_viverrini_data.html . Clustering of orthologous genes All proteins predicted from the gene set of O. viverrini were clustered with orthologous in C. sinensis [13] , S. haematobium [9] , S. japonicum [10] and S. mansoni [11] , and the tapeworms Echinococcus multilocularis , Echinococcus granulosus and Taenia solium [21] using OrthoMCL ( http://orthomcl.org/orthomcl/ ). Phylogenetic analyses To assess the expansion of the protein families in O. viverrini relative to the other parasitic flukes, amino sequence data relating to specific protein families were extracted, aligned using the program MUSCLE ( https://www.ebi.ac.uk/Tools/msa/muscle/ ) and manually verified. To assess evolutionary relationships between and among the protein families, phylogenetic trees were constructed by Bayesian inference using the program Mr Bayes v. 3.1.2 ( http://mrbayes.sourceforge.net/ ) employing the Monte Carlo Markov chain method (nchains=4) over 1,000,000 tree-building generations, with every 100th tree being saved; 25% of the first saved trees were discarded to ensure stabilization of the nodal split frequencies, and consensus trees for each protein family were constructed from all remaining trees, with the nodal support for each clade expressed as a posterior probability value. The consensus trees were labelled using the program Figtree v.1.4 ( http://tree.bio.ed.ac.uk/software/figtree/ ). Motif logos across conserved domains were drawn using a sequence logo generator tool ( http://weblogo.berkeley.edu/ ). Accession codes: Sequence data for Opisthorchis viverrini have been deposited in the GenBank/EMBL/DDBJ nucleotide core database under the accession code JACJ00000000 and using the gene codes T2650000001 to T2650016380. How to cite this article: Young, N. D. et al. The Opisthorchis viverrini genome provides insights into life in the bile duct. Nat. Commun. 5:4378 doi: 10.1038/ncomms5378 (2014).